Scalable organocatalytic asymmetric Strecker reactions catalysed by a chiral cyanide generator The Strecker synthesis is one of the most facile methods to access racemic α-amino acids. However, feasible catalytic asymmetric Strecker reactions for the large-scale production of enantioenriched α-amino acids are rare. Here we report a scalable catalytic asymmetric Strecker reaction that uses an accessible chiral variant of oligoethylene glycol as the catalyst and KCN to generate a chiral cyanide anion. Various α-amido sulphone substrates (alkyl, aryl and heteroaryl) can be transformed into the optically enriched Strecker products, α-aminonitriles, with excellent yields and enantioselectivities. Moreover, the robust nature of the catalyst enables a ‘one-pot’ synthesis of enantiomerically pure α-amino acids starting from α-amido sulphones and simple catalyst recycling. These features can make this protocol easily adaptable to the practical synthesis of unnatural α-amino acids. αc-Amino acids are the building blocks of proteins and are widely used as components of pharmaceutically active molecules and chiral catalysts [1] . In particular, synthetic unnatural α-amino acids have had a significant role in the area of peptide research. They have been used extensively in peptide analogues to limit conformational flexibility, enhance enzymatic stability, and improve pharmacodynamics and bioavailability [2] . The Strecker synthesis [3] —the reaction of an imine or imine equivalent with hydrogen cyanide, followed by nitrile hydrolysis—is a standard method for producing α-amino acids [4] , [5] , [6] , [7] . Although there is already a number of useful catalytic asymmetric variants showing high catalyst efficiency [8] , [9] , [10] , [11] , [12] , [13] , [14] , [15] , [16] , [17] , the limited utility of existing catalytic methods may be due to several important factors, including the relatively complex and precious nature of the catalysts, and the use of hazardous cyanide sources (for example, HCN, acetone cyanohydrin or trimethylsilyl cyanide) in super-stoichiometric amounts, preventing their practical application to large-scale processes. Moreover, it has often been observed that direct hydrolysis of optically active α-aminonitriles can result in deterioration of optical purity of the amino acid products [18] . Therefore, it is still highly desirable to develop a more practical and general catalytic system, which includes a convenient cyanide source (for example, KCN), a broader scope of substrates, easily available and recyclable catalysts, and mild reaction conditions and racemization-free hydrolysis conditions. Recently we have developed a highly efficient methodology for nucleophilic substitution reactions with various potassium salts, using oligoethylene glycols as a new type of a multifunctional promoter [19] , [20] . The multifunctional activation mode of a polyethylene glycol renders unprecedented selectivity, activity and efficiency to various inorganic salts. Further investigation into the asymmetric application of this protocol revealed that a chiral variant of oligoethylene glycols could be applied as a new structural motif of a chiral promoter system, which is highly accessible from an axially chiral 1,1′-binaphthol backbone and polyethylene glycols ( Fig. 1 ) [19] , [21] . Using this catalytic system, we have reported a highly enantioselective desilylative kinetic resolution of a variety of silyl-protected secondary alcohols with potassium fluoride [21] . Under the reaction conditions, this type of a promoter brings insoluble potassium salts into the organic solution by forming a chiral ion pair. This resulting chiral ion pair can then mediate an asymmetric reaction. Therefore, we presumed that our chiral anion generator can be applied to catalytic enantioselective Strecker synthesis by generating a chiral cyanide anion to provide a more general and practical method to access enantiomerically pure non-natural amino acids. 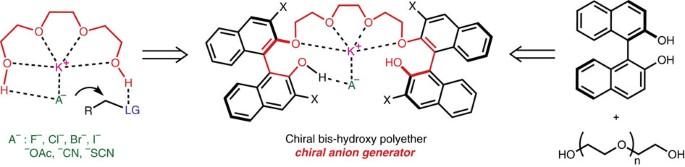Figure 1: Chiral bis-hydroxy polyether as a chiral anion generator. LG, leaving group; X, halogen atom. Figure 1: Chiral bis-hydroxy polyether as a chiral anion generator. LG, leaving group; X, halogen atom. Full size image Here we report a new organocatalytic, highly enantioselective Strecker protocol, using 3,3′-diiodine-substituted BINOL (1,1'-bi-2,2'-naphthol)-based catalyst 1a , which enables the direct use of a broad scope of α-amido sulphones [22] , [23] , [24] , as stable precursors of the corresponding sensitive and unstable N -carbamoyl aldimines, and potassium cyanide as an inexpensive, safe and convenient cyanide source in an organic medium. In particular, the structural robustness of the catalyst enables a ‘one-pot’ synthesis of enantiomerically pure non-natural α-amino acids and easy catalyst recycling. Reaction design To extend the application of our polyether-tethered chiral catalyst ( Fig. 1 ), we first examined a Strecker reaction of the Boc ( tert -butyloxycarbonyl)-protected imine 2a (ref. 25 ) with KCN in the presence of 10 mol% of ( R )-1a in toluene at 0 °C (conditions (a) in Fig. 2 ). However, the reaction proceeded very sluggishly to afford the desired α-amino nitrile product ( R )- 3a with disappointing enantioselectivity (69% enantiomeric excess (ee), 24% yield). However, interestingly, when using the α-amido sulphone 4a , which is a stable synthetic precursor of imine 2a , the same reaction proceeded smoothly, affording the product with an excellent yield and enantioselectivity (93% ee, conditions (c) in Fig. 2 ). It should be noted here that the preparation of α-aminonitriles from α-amido sulphones has recently been reported [26] , [27] , [28] , [29] . However, the enantioselective versions using asymmetric phase transfer catalysts [27] , [28] and quinine as a chiral base [29] showed a limited substrate scope and/or only moderate enantioselectivity. We next conducted the Strecker reaction of the imine 2a with HCN as a cyanide source in the presence of the catalyst ( R )-1a . Even after 60 h, we could obtain only a trace amount of α-amino nitrile ( R )- 3a (<5%) with a very low ee value (34% ee; conditions (b) in Fig. 2 ). These results suggested that the interaction between the sulphinate group (−SO 2 Ph) and the catalyst is very important for catalyst performance. 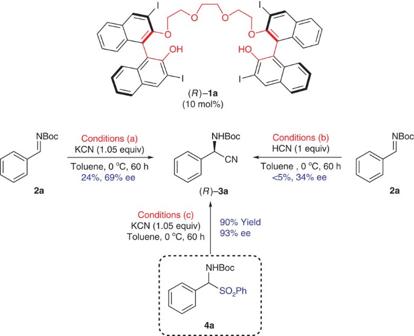Figure 2: Strecker synthesis using the chiral anion generator1a. Boc,tert-butyloxycarbonyl. Figure 2: Strecker synthesis using the chiral anion generator 1a . Boc, tert -butyloxycarbonyl. Full size image Optimization of the reaction conditions Next, we screened the catalytic efficiency of a variety of chiral BINOL-based bis(hydroxy) polyethers 1 to shed light on the relationship between the structures of catalysts and reaction outcomes. As shown in Fig. 3 , the observed relationship between the structure and catalytic performance was almost the same as that observed previously in the desilylative kinetic resolution of racemic alcohols with KF ( [21] ). Thus, only those catalysts having halogen substituents at the 3,3′-position on the BINOL group exhibited catalytic activity ( Fig. 3a ). When catalysts ( R )-1b and ( R )-1c having no halogen substituent at the 3,3′-position (R=H or Ph) were employed, only a very low level of conversion and enantioselectivity were observed. Moreover, a dramatic enhancement in both activity and enantioselectivity was observed when switching from chlorine to iodine (from 38 to 93% ee). Thus, the best enantioselectivity was obtained when the 3,3′-diiodo-substituted chiral BINOL catalyst 1a was used. Higher activity and greater stereoselectivity of 3,3′-diiodo-substituted catalyst 1a than those having chlorine or bromine substituents at 3,3′-position can be explained by the greater polarizability of the iodine atoms compared with those of the chlorine and bromine atoms, which allows it to more strongly coordinate to the potassium cation (see ref. 21 for X-ray crystal structure of the catalyst–KF complex). In addition to this strong coordination of the iodine atom to the potassium cation, the larger steric size of iodine might also influence the chiral environment of the transition state, resulting in the observed enhancement of enantioselectivity. As expected, the ether chain length, which is responsible for the formation of a suitable chiral coordination cage with a potassium cation, was also shown to have a crucial role in the performance of the catalyst. The catalyst having three ether units (–(OCH 2 CH 2 ) 3 –) was shown to be a much more effective catalyst than other catalysts bearing longer (4-ether units; 1g ; 0% ee) or shorter (2-ether units; 1f ; 9% ee) sequences of ether units ( Fig. 3b ). As shown in Fig. 3c , it was also observed that the terminal free hydroxyl group at the 2,2′-position of the BINOL backbone has an essential role in maintaining the superior catalytic performance of the multifunctional catalyst. Mono- O -methyl protected catalyst ( R )-1h displayed significantly lower efficiency (typically <50% conversion and 51% ee). Moreover, di- O -methyl protected catalyst ( R )-1i was completely inactive in the same reaction conditions. This observation suggests that a hydrogen-bonding interaction between the free hydroxyl groups of catalyst and the amido sulphone, activating the imine precursor and rigidifying the transition structure, has a key role in this highly stereoselective transformation. Notably, we found that the phenolic proton of the catalyst is not transferred to the product; when using the deuterated amido sulphone as the substrate, only deuterated aminonitrile was observed ( Supplementary Fig. S1 ). 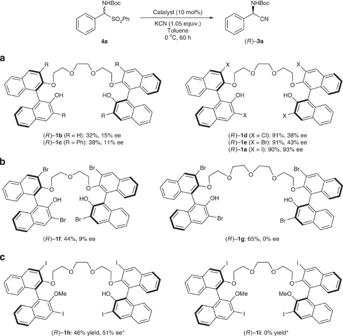Figure 3: Influence of the catalyst structure on the reaction. (a) Effects of the substituents at the 3,3′-position on the BINOL group for the catalyst performance. (b) Effects of the ether chain length for the catalyst performance. (c) Effects of phenolic protons for catalyst performance. *The reactions were carried out at room temperature for 36 h. Figure 3: Influence of the catalyst structure on the reaction. ( a ) Effects of the substituents at the 3,3′-position on the BINOL group for the catalyst performance. ( b ) Effects of the ether chain length for the catalyst performance. ( c ) Effects of phenolic protons for catalyst performance. *The reactions were carried out at room temperature for 36 h. Full size image Substrate scope of the reaction Finally, under optimized conditions, a variety of aldimines were subjected to this protocol. As shown in Fig. 4 , a variety of α-amido sulphones, 4a–4o , were smoothly converted to the corresponding amino nitriles ( R )- 3 with excellent yields and enantioselectivities. The opposite enantiomer of amino nitriles ( S )- 3 were also obtained by employing the catalyst ( S )-1a . In general, higher enantioselectivity was obtained for electron-rich aromatic aldimines. In the case of the electron-deficient aromatic substrates 4c and 4d , the reactions were conducted at a lower temperature (−20 °C, >91% ee) to obtain higher enantioselectivity. Heteroaromatic substrates such as 3-pyridyl ( 4k ) and 3-thienyl ( 4l ) also gave satisfactory yields and enantioselectivities. In addition, secondary and tertiary aliphatic substrates provided the desired amino nitriles, ( R )- 3m and ( R )- 3n , with high yields and enantioselectivities. However, in the case of primary alkyl-substituted aminonitrile ( 3o ), moderate yield and low enantioselectivity were observed, due to the imine–enamine tautomerism. However, fortunately, primary alkyl-substituted aminonitrile 3o showed an enantiomeric enrichment upon a simple crystallization similar to most of other α-aminonitriles (see high-performance liquid chromatography (HPLC) spectra of ( R )- 3o in Supplementary Fig. S16 ). Finally, it should be noted that only one equivalent of KCN was required to obtain the best catalytic results. The use of excess amounts (2 equiv.) of KCN gave the inferior results (for example, 89% ee for ( R )- 3a ) due to the background reaction (see Supplementary Table S1 for details of background reaction experiments). 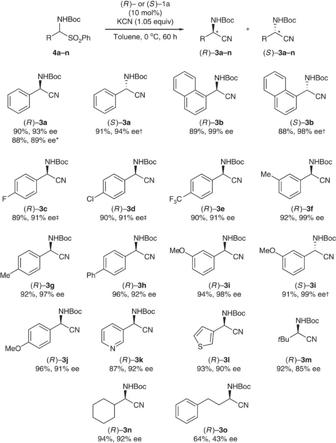Figure 4: Scope of the enantioselective Strecker reaction of α-amido sulphones with KCN. Unless otherwise indicated, the reactions were carried out with4(0.1–0.5 mmol), 1.05 equiv. of KCN, and(R)-1acatalyst (10 mol%) in toluene at 0 °C. * Two equivalents of KCN were used. †(S)-1acatalyst was used. ‡ The reaction was carried out using 20 mol% of catalyst at −20 °C for 84 h. Figure 4: Scope of the enantioselective Strecker reaction of α-amido sulphones with KCN. Unless otherwise indicated, the reactions were carried out with 4 (0.1–0.5 mmol), 1.05 equiv. of KCN, and ( R )-1a catalyst (10 mol%) in toluene at 0 °C. * Two equivalents of KCN were used. † ( S )-1a catalyst was used. ‡ The reaction was carried out using 20 mol% of catalyst at −20 °C for 84 h. Full size image One-pot syntheses of α-amino acids Moreover, the present protocol was successfully applied to the synthesis of five different non-proteinogenic amino acids, which are topically interesting subunits of pharmaceutically active agents. Very importantly, the robust nature of catalyst 1 allowed for a highly practical ‘one-pot’ process for the preparation of enantiomerically pure non-natural α-amino acids and easy catalyst recycling ( Fig. 5 ). Under the present catalytic protocol (10 mol% of ( R )-1a , 1.05 equiv. of KCN, 0 °C, 60 h), Boc-protected α-amido sulphones 4a , 4b , 4i , 4m and 4n (4–10 mmol scale) were smoothly transformed into the corresponding α-aminonitriles ( R )- 3a , 3b , 3i , 3m and 3n . Without any extra separation of α-amino nitrile and the catalyst, the crude product mixture was then subjected to the hydrolysis conditions (6 N HCl, 100 °C) [26] . The water-insoluble organocatalyst 1a could simply be recovered from the hydrolysis product mixture by simple phase separation (recovery yield >95%), allowing for repeated recycling (for the catalyst recycling experiment, see Supplementary Methods and Supplementary Figs S23–S24 ). Evaporation of the aqueous solution and recrystallization of the residue with water or i -PrOH afforded the HCl salt of enantiomerically pure amino acids, such as ( R )-phenylglycine (( R )- 6a ; 65%, >99% ee), ( R )-1-naphthylglycine (( R )- 6b ; 55%, >99% ee), ( R )- m -methoxyphenylglycine (( R )- 6i ; 65%, >99% ee), ( R )- tert -leucine (( R )- 6m ; 54%, >99% ee) and ( R )-cyclohexylglycine (( R )- 6n ; 66%, >99% ee). 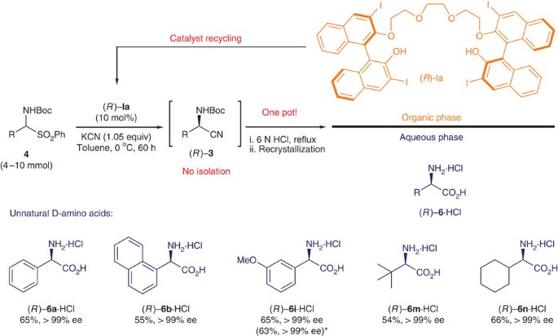Figure 5: Gram-scale one-pot synthesis of some pharmacologically important non-proteinogenic amino acids and catalyst recycling. *Using the recovered catalyst(R)-1a Figure 5: Gram-scale one-pot synthesis of some pharmacologically important non-proteinogenic amino acids and catalyst recycling. *Using the recovered catalyst ( R )-1a Full size image The detailed reaction mechanism and the origin of the observed enantioselectivity are as yet unclear. However, all the experimental results discussed above shed some light on a possible reaction mechanism ( Fig. 6a ) involving the following: initial simultaneous activation of KCN and amido sulphone by the catalyst, elimination of the sulphinate from amido sulphone by potassium cyanide to generate a catalyst-bound imine or iminium/cyanide pair and subsequent cyanation of the activated imine to provide the enantiomerically enriched α-aminonitrile. According to the proposed mechanism, the cyanide anion will have sequential roles of a base and a nucleophile. This is also consistent with the fact that the reaction performed with only 1.05 equiv. of KCN afforded the expected α-aminonitrile ( R )- 3a in 90% yield and 93% ee. More importantly, according to this mechanism, potassium benzenesulphinate has a crucial role in generating the suitable chiral cage in the transition state. 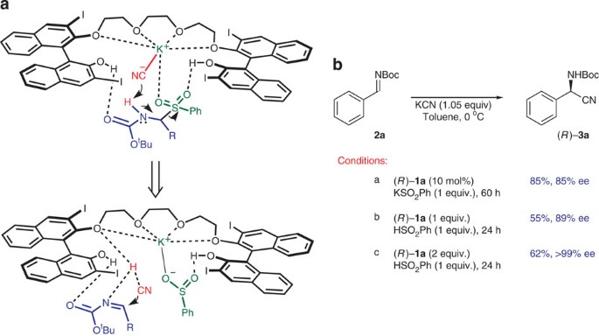Figure 6: Reaction mechanism. (a) A plausible reaction transition state. (b) Critical effects of the additional sulphinate anion. Figure 6: Reaction mechanism. ( a ) A plausible reaction transition state. ( b ) Critical effects of the additional sulphinate anion. Full size image To support this suggested reaction mechanism, we carried out control experiments by varying reaction conditions. Imine 2a , which was not reactive under the reaction conditions with KCN, was converted to the desired product ( R )- 3a with 85% yield and 85% ee in the presence of potassium benzenesulphinate (1 equiv. ; conditions (a) in Fig. 6b ). Furthermore, to resemble the reaction conditions with N -Boc-protected sulphone 4a and KCN, we subjected imine 2a to the reaction using a mixture of KCN and phenylsulphinic acid [30] from which HCN and potassium benzenesulphinate can be generated in situ . An excellent level of enantioselectivity (up to >99% ee) was obtained by using more than one equivalent of the catalyst ( R )-1a (conditions (b) and (c) in Fig. 6b ). These results again suggest the importance of sulphinate anion in the enantio-determining step, which might be ascribed to the ionic and hydrogen-bonding interactions between the catalyst, imine, HCN and potassium benzenesulphinate. In conclusion, we have successfully developed a new catalytic asymmetric method for the syntheses of highly enantiomerically enriched non-natural amino acids using a highly enantioselective 3,3′-diiodine-substituted BINOL-based catalyst 1a to control the key hydrocyanation step in the asymmetric Strecker reaction. In the presence of highly accessible catalyst 1a , a variety of α-amido sulphones were converted to the corresponding amino nitriles with potassium cyanide in high yields and enantioselectivity. Enantiomerically pure α-amino acids were then easily obtained by simple hydrolysis of the enantioenriched amino nitriles and a single recrystallization step. This study represents a new approach to asymmetric Strecker-type reactions, which holds the following distinctive practical advantages: it avoids the use of highly toxic HCN and, moreover, it requires only one equivalent of KCN; it enables the direct use of a broad scope of α-amido sulphones (alkyl, aryl and heteroaryl) and, thus, it does not require extra isolation of the labile imine intermediate; in particular, the structural simplicity and robustness of the catalyst enable ‘one-pot’ synthesis of enantiomerically pure non-natural α-amino acids and simple recovery of the catalyst. All of these factors can render this protocol easily adaptable to the large-scale synthesis of non-natural amino acids. Materials and characterization All starting materials and anhydrous solvents were obtained from commercial suppliers and used without purification. α-Amido sulphones [25] 4 and racemic amino nitriles [26] 3 were obtained according to literature procedures. Thin-layer chromatography (TLC) was performed on silica gel plates (Merck, Kieselgel 60 F254, 0.25 mm) or NH-silica gel plates (Fuji Silysia, NH TLC plate). For preparative TLC, Merck pre-coated PLC plates (silica gel 60 F254, 0.5 mm) were used. The chromatographic purification of the products was carried out by using Merck silica gel 60 (230–400 mesh) or NH silica gel (Fuji Silysia, 100–200 mesh). The 1 H NMR (300 and 500 MHz) and 13 C NMR (75 and 125 MHz) spectra were recorded on Varian 300 or Varian 500 spectrometers. Chemical shifts are reported in ppm downfield from tetramethylsilane or sodium 3-(trimethylsilyl)tetradeuteriopropionate as an internal standard in organic NMR solvents or D 2 O, respectively. The HPLC analyses for the determination of the ee of the products were performed on a Varian Pro Star Series instrument equipped with an isostatic pump using a CHIRALCEL Column (250 × 4.6 mm), or on a YoungLin instrument equipped with an isostatic pump using a Sumichiral column OA-5,000 (250 × 4.6 mm). Gas chromatography analyses for the determination of the ee of the products were performed on a Younglin YL6100GC instrument using an RT-BetaDEX-sm chiral column. The infrared spectra were obtained using a Bruker Vertex 70 spectrometer with the MIRacle Micro ATR accessory. The high-resolution mass spectra were measured using fast atom bombardment method on a Jeol JMS-700 Mstation. The melting points were determined by using a Buchi B-540 melting point apparatus and are uncorrected. The optical rotation was measured using a PerkinElmer Polarimeter 343 plus. Preparation and characterization of chiral catalysts 1 Preparation and characterization of catalysts 1 ( [21] ) are included in Supplementary Methods and Supplementary Figs S2–S11 . Procedure for the catalytic asymmetric Strecker reactions In a 10-ml flask, α-amido sulphone 4 (0.50 mmol), KCN (0.525 mmol) and ( R )-1a (59.5 mg, 0.05 mmol, 10 mol%) were added. The flask was evacuated and then purged with Ar gas. To the Ar-purged flask, 6 ml of anhydrous toluene as a solvent was added through the septum, and the reaction mixture was stirred at 0 °C. Upon completion of the reaction (ca. 60 h), the reaction mixture was filtered and the filter cake (KSO 2 Ph) was washed with toluene. The filtrate was then concentrated under reduced pressure (caution: toxic HCN vapour can evolve, use a well-ventilated fume hood). Purification of the residue by flash column chromatography on silica gel (acetone/hexanes/NEt 3 =1:5:0.025 as eluent) gave the corresponding α-aminonitrile ( R )- 3 . α-Aminonitriles were characterized by 1 H, 13 C NMR and infrared ( Supplementary Figs S12–S13 ), and the enantiomeric excesses were determined by chiral HPLC analysis ( Supplementary Figs S14–S17 and S25 ). Racemic α-aminonitriles 3a , 3b , 3d , 3f , 3g , 3i , 3j and 3m – 3o are known compounds in literature, and spectroscopical data are consistent with previously reported values [26] , [31] . The absolute configurations of 3a , 3b , 3d , 3f , 3g , 3i , 3j and 3m – 3o were determined by comparison of the retention time of HPLC or gas chromatography with the literature data [27] , [29] , [32] , [33] . The absolute configurations of 3c , 3e , 3h , 3k and 3l were assigned by analogy. Typical procedure for the one-pot synthesis of ( R )-6a·HCl In a 100-ml flask, α-amido sulphone 4a (1.39 g, 4 mmol), KCN (0.27 g, 4.2 mmol, 1 equiv.) and ( R )-1a (0.48 g, 0.4 mmol, 10 mol%) were added. The flask was evacuated and then purged with Ar gas. To the Ar-purged flask, 48 ml of anhydrous toluene as a solvent was added through the septum, and the reaction mixture was stirred at 0 °C. Upon completion of the reaction (ca. 60 h), the reaction mixture was filtered through a membrane and the filter cake (KSO 2 Ph) was washed with toluene. To the filtrate, 50 ml of 6 N HCl was added and the mixture was heated to 65 °C for 2 h. After cooling the reaction mixture to room temperature, the organic layer was separated and the aqueous layer was extracted with toluene (2 × 25 ml). The organic layer was dried over Na 2 SO 4 , filtered and evaporated to give an ivory white organocatalyst ( R )-1a (0.46 g) in almost pure form. The recovered catalyst 1a can be further purified by washing with methanol. The aqueous layer was heated under reflux for 3 h, cooled to room temperature and washed with EtOAc (2 × 25 ml). After concentration of the aqueous layer under vacuum, recrystallization of the residue from i -PrOH afforded the enantiomerically pure phenylglycine as hydrochloride salt ( R )- 6a ·HCl (0.49 g, 65% yield, >99% ee). Analytical data of ( R )- 6a ·HCl, ( R )- 6b ·HCl, ( R )- 6i ·HCl, ( R )- 6m ·HCl and ( R )- 6n ·HCl are included in Supplementary Figs S18–S22 . How to cite this article: Yan, H. et al . Scalable organocatalytic asymmetric Strecker reactions catalysed by a chiral cyanide generator. Nat. Commun. 3:1212 doi: 10.1038ncomms/2216 (2012).